Interplay between enterobactin, myeloperoxidase and lipocalin 2 regulatesE. colisurvival in the inflamed gut During an inflammatory response in the gut, some commensal bacteria such as E. coli can thrive and contribute to disease. Here we demonstrate that enterobactin (Ent), a catecholate siderophore released by E. coli , is a potent inhibitor of myeloperoxidase (MPO), a bactericidal enzyme of the host. Glycosylated Ent (salmochelin) and non-catecholate siderophores (yersiniabactin and ferrichrome) fail to inhibit MPO activity. An E. coli mutant (Δ fepA) that overproduces Ent, but not an Ent-deficient double mutant (Δ aroB/ Δ fepA) , inhibits MPO activity and exhibits enhanced survival in inflamed guts. This survival advantage is counter-regulated by lipocalin 2, a siderophore-binding host protein, which rescues MPO from Ent-mediated inhibition. Spectral analysis reveals that Ent interferes with compound I [oxoiron, Fe(IV)=O] and reverts the enzyme back to its native ferric [Fe(III)] state. These findings define a fundamental mechanism by which E. coli surpasses the host innate immune responses during inflammatory gut diseases and gains a distinct survival advantage. The mammalian intestine harbours a community of bacteria collectively known as the microbiota. Both the host and the microbiota depend on and compete for common nutrients, such as the essential trace transition metal iron, for their proliferation and biologic functions. In the host, the majority of circulating iron is bound to host proteins, resulting in low free-iron availability (10 −24 M), which functions as a ‘natural antibiotic/nutritional immunity’ mechanism for controlling bacterial growth [1] , [2] , [3] . The bacteria circumvent low iron levels in the host by expressing a suite of siderophores with high affinity for iron. Enterobactin (Ent), a prototypical and conserved siderophore, has an unmatched affinity for iron ( K d of 10 −35 M at physiologic pH) [4] , allowing Ent to chelate iron from iron-binding host proteins such as ferritin and transferrin. The monomeric form of Ent, designated 2,3-dihydroxybenzoic acid (DHBA), is produced by Brucella abortus under conditions of low iron availability [5] . Previous studies have demonstrated that pathogens that synthesize defective siderophores are less virulent [6] , [7] . In fact, many pathogens sense the low iron levels in the host (for example, hypoferremia of inflammation) as an environmental cue to trigger synthesis of virulence factors [3] , [8] . Further, iron acquisition by siderophores plays a significant role in extraintestinal pathogenic E. coli virulence [9] . Neutrophils are the most abundant white blood cells in circulation and are the first responder cell type during infection, inflammation and injury. Myeloperoxidase (MPO, Enzyme Commission: 1.11.2.2), a haem protein and a marker of neutrophils, requires Fe +3 for its bioactivity. During respiratory burst, MPO uses H 2 O 2 and halide ions to generate hypochlorous acid, a potent oxidizing and antimicrobial agent [10] . Lactoperoxidase (LPO, Enzyme Commission: 1.11.1.7), a similarly haem-containing milk protein, shares a number of overlapping properties with MPO [11] . In neutrophils, MPO is a companion of the siderophore-binding protein lipocalin 2 (Lcn2, also known as neutrophil gelatinase-associated lipocalin). Lcn2 acts as part of the first line of defence against invading microbes by chelating bacterial siderophores with high affinity (0.4 nM) [1] , depriving them of iron. Although Lcn2 has no measurable affinity for Fe +3 alone, it can bind to siderophores alone or to Fe +3 -bound siderophores (for example, Ent or Fe +3 -Ent) [12] . Gut bacterial dysbiosis is associated with a number of gastrointestinal disorders including human immunodeficiency virus enteropathy [13] , necrotizing enterocolitis [14] , Crohn’s disease [15] , irritable bowel syndrome [16] , inflammation-associated enterotype [17] , antibiotic treatment [18] , enteropathogen infection, chemical- and genetically induced colitis [19] and protozoan parasite infection [20] . One of the potential mechanisms by which Enterobacteriaceae flourish despite the inflammatory milieu is through utilization of stable reactive oxygen and nitrogen species produced as by-products of the host innate inflammatory response as electron acceptors, therefore supporting their growth and anaerobic respiration [21] , [22] , [23] . In this study, we show that the bacterial siderophore Ent and its monomeric form DHBA inhibit MPO/LPO activity in vitro and inhibit MPO activity in the inflamed gut. Inhibition of MPO activity by Ent confers a distinct survival advantage and permits enhanced colonization by E. coli in the inflammatory state. Elucidation of possible underlying mechanisms via spectral analysis using LPO–H 2 O 2 as a model system reveals that Ent acts as a potent, fast-acting suicide substrate that prevents hypohalous acid formation in the peroxidase-catalysed reaction. Collectively, our study describes a novel mechanism that promotes survival and growth of E. coli , a well-known opportunistic pathogen in a variety of chronic intestinal diseases associated with microbiotal dysbiosis. Apo-enterobactin is a potent inhibitor of MPO activity Microbiotal dysbiosis is commonly observed in several types of inflammatory bowel diseases (IBDs). Specifically, IBD is associated with a bloom in bacterial species belonging to the family Enterobacteriaceae (for example, E. coli) , class Gammaproteobacteria , within the phylum proteobacteria. It has been shown that E. coli thrives in inflammatory conditions by expressing several genes that confer a survival advantage. In this study, we asked whether the Fe +3 -chelating siderophore, apo-Ent (Fe +3 free), could affect the bioactivity of the dimeric haem protein MPO, which requires Fe +3 for its function. As shown in Fig. 1a , cyclic apo-Ent inhibited MPO activity in a dose-dependent manner. Specifically, apo-Ent at 1.0 and 30 μM concentration inhibited 50 and 80% of MPO activity, respectively. DHBA, an intermediate in the Ent biosynthesis with lower affinity for Fe +3 than Ent, also inhibited MPO activity in a dose-dependent manner, although to a lesser extent than Ent. The dose–response curve and time–kinetic response of MPO inhibition by Ent and DHBA revealed that Ent is a more potent and fast-acting inhibitor of MPO activity than DHBA ( Fig. 1a,b ). Nevertheless, both Ent and DHBA are more potent and fast-acting inhibitors of MPO activity than 4-aminobenzoic hydrazide (ABAH), a known inhibitor of MPO [24] . In a similar fashion, Ent and DHBA inhibited monomeric haem protein LPO activity in a dose- and time-dependent manner ( Supplementary Fig. 1 ). Surprisingly, DHBA was found to be more potent than Ent in inhibiting LPO activity ( Supplementary Fig. 1A ). The inhibitory effect of Ent on MPO activity was observed even after the initiation of the MPO reaction and over a range of temperatures and pH ( Supplementary Fig. 2A–C ). To determine whether inhibition of MPO or LPO is an inherent property of all siderophores or is specific to Ent, we tested MPO and LPO inhibitory activity of salmochelin, yersiniabactin and ferrichrome, which showed only ∼ 13, ∼ 5 and ∼ 0.5% MPO inhibitory activity, respectively, even at concentrations 50 times greater than Ent ( Supplementary Fig. 3A–C ). In the same way, these siderophores were weak inhibitors of LPO activity ( Supplementary Fig. 3D–F ). Taken together, these observations suggest that MPO and LPO inhibitory activity is relatively more specific to Ent. 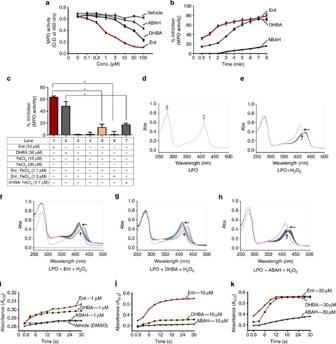Figure 1: AferricE. colisiderophore enterobactin (Ent) inhibits MPO activity. Ent, DHBA or ABAH was pre-incubated at the below indicated final concentrations, with 100 mU of MPO for 10 min and then MPO activity was quantitatively measured using guaiacol (100 mM) and H2O2(6.7 × 10−3%). Line graph represents (a) dose- (0.1–100 μM) and (b) time (0.5–8 min)-dependent inhibition of MPO activity by 30 μM of Ent, DHBA or ABAH. (c) Ent or DHBA was pre-incubated with FeCl3for 1 min and subsequently incubated with MPO for 10 min. Bar graph represents percent inhibition of MPO activity by apo- or Fe+3-saturated Ent or DHBA. Assays were carried out in 96-well plates in triplicate with appropriate vehicles/buffers throughout the study. (d–h) To perform spectral analysis, LPO (2.6 nM, in 0.1 M phosphate buffer) was incubated with various concentrations of Ent, DHBA or ABAH for 1 min. The reaction was initiated by the addition of 30 μM H2O2. Spectra (250–500 nm) were recorded up to 3 min. Each spectrum is an average of three scans taken in 1.0 s. Image displays the spectra of (d) LPO alone, (e) LPO+H2O2, (f) LPO+Ent (30 μM)+H2O2, (g) LPO+DHBA (30 μM)+H2O2and (h) LPO+ABAH (30 μM)+H2O2. (i–k) Time-dependent change in the absorbance spectra of LPO at 412 nm at various concentrations of ABAH, Ent and DHBA. Arrows indicate the direction of spectral changes, that is, conversion of oxoiron [Fe(IV)=O] to the native form [Fe(III)]. Results are expressed as mean±s.e.m. and are representative of six independent experiments (a–c). Data represent one of three similar experiments (f–k).*P<0.05, unpairedt-test. Figure 1: Aferric E. coli siderophore enterobactin (Ent) inhibits MPO activity. Ent, DHBA or ABAH was pre-incubated at the below indicated final concentrations, with 100 mU of MPO for 10 min and then MPO activity was quantitatively measured using guaiacol (100 mM) and H 2 O 2 (6.7 × 10 −3 %). Line graph represents ( a ) dose- (0.1–100 μM) and ( b ) time (0.5–8 min)-dependent inhibition of MPO activity by 30 μM of Ent, DHBA or ABAH. ( c ) Ent or DHBA was pre-incubated with FeCl 3 for 1 min and subsequently incubated with MPO for 10 min. Bar graph represents percent inhibition of MPO activity by apo- or Fe +3 -saturated Ent or DHBA. Assays were carried out in 96-well plates in triplicate with appropriate vehicles/buffers throughout the study. ( d – h ) To perform spectral analysis, LPO (2.6 nM, in 0.1 M phosphate buffer) was incubated with various concentrations of Ent, DHBA or ABAH for 1 min. The reaction was initiated by the addition of 30 μM H 2 O 2 . Spectra (250–500 nm) were recorded up to 3 min. Each spectrum is an average of three scans taken in 1.0 s. Image displays the spectra of ( d ) LPO alone, ( e ) LPO+H 2 O 2 , ( f ) LPO+Ent (30 μM)+H 2 O 2 , ( g ) LPO+DHBA (30 μM)+H 2 O 2 and ( h ) LPO+ABAH (30 μM)+H 2 O 2 . ( i – k ) Time-dependent change in the absorbance spectra of LPO at 412 nm at various concentrations of ABAH, Ent and DHBA. Arrows indicate the direction of spectral changes, that is, conversion of oxoiron [Fe(IV)=O] to the native form [Fe(III)]. Results are expressed as mean±s.e.m. and are representative of six independent experiments ( a – c ). Data represent one of three similar experiments ( f – k ). * P <0.05, unpaired t -test. Full size image During conditions of iron scarcity, bacteria drastically upregulate expression of siderophores to acquire this essential metal. After binding Fe +3 in the stoichiometry of 1:1, Ent is internalized by bacteria via the FepA receptor. Next, we asked whether Fe +3 -bound Ent possesses MPO inhibitory activity. We incubated Fe +3 (sourced from FeCl 3 ) with apo-Ent in a 1:1 and 3:1 ratio at 37 °C for 5 min. Interestingly, Fe +3 -Ent in a ratio of 3:1 completely failed to inhibit MPO activity, whereas Fe +3 -Ent in the 1:1 ratio was still able to inhibit MPO activity to some extent ( Fig. 1c ). FeCl 3 alone at 30 μM did not influence the MPO-catalysed reaction. Similarly, Fe +3 -DHBA (1:1) failed to inhibit MPO activity ( Fig. 1c ), suggesting that the inhibitory effect of Ent on these iron-containing enzymes require its Fe +3 -free form. To delineate the possible underlying mechanism of Ent-induced inhibition of MPO activity, we performed spectral analysis of a peroxidase-catalysed reaction with H 2 O 2 in the presence or absence of apo forms of Ent and DHBA using LPO. LPO exhibits similar activity to MPO but is more affordable (than MPO) and therefore practical for usage in spectral analyses. Before starting spectral analysis, we monitored the characteristic spectra of LPO, which showed λ max at 412 nm ( Fig. 1d ). Upon addition of H 2 O 2 (30 μM), LPO was converted into a redox intermediate with λ max at ∼ 430 nm, which is characteristic of the compound II (Fe(IV)=OH-porphyrin) ( Fig. 1e ). In the presence of Ent (30 μM), H 2 O 2 mediated a shift in the Soret band and reverted back (denoted by arrows) to 412 nm within seconds, suggesting the regeneration of native LPO ( Fig. 1f ). Similarly, DHBA at 30 μM completely reverted the shifted peak to 412 nm within seconds ( Fig. 1g ). In agreement with our in vitro data, ABAH (30 μM) did not completely revert the H 2 O 2 -induced shift in LPO spectra ( Fig. 1h ), suggesting it is a weaker inhibitor than Ent or DHBA ( Fig. 1a,b ). Furthermore, a dose-dependent response of Ent, DHBA and ABAH on the regeneration of native LPO revealed that both apo-Ent and DHBA are more potent and fast-acting suicide substrates than ABAH ( Fig. 1i–k ). The haem [Fe(III)] in LPO participates in a redox reaction, and is converted to oxoiron [Fe(IV)=O], also known as ‘compound I’, upon the addition of H 2 O 2 . In the presence of a halide ion, compound I is reduced back to its ferric state, [Fe(III)] and this results in hypohalous acid formation, a potent bactericidal agent. As we observed in our spectral analyses, Ent and DHBA reduced the oxoiron [Fe(IV)=O] to the native enzyme [Fe(III)], effectively preventing the formation of hypohalous acid. There was no change in the spectra of LPO observed upon addition of Ent, DHBA or ABAH in the absence of H 2 O 2 , suggesting that they do not directly interact with Fe +3 in the haem moiety ( Supplementary Fig. 4A–D ). Collectively, these results demonstrate that both Ent and DHBA are fast-acting suicide substrates that accelerate native peroxide formation and consequently prevent the generation of the potent oxidizing antimicrobial agent hypohalous acid. E. coli -produced enterobactin inhibits MPO activity Host inflammatory conditions are generally characterized by hypoferremia [25] , an environmental signal that prompts bacteria to overexpress siderophores [3] . To address whether Ent-expressing bacteria can exert MPO inhibitory activity, we took advantage of E. coli mutants that either overproduce Ent (Δ fepA ) or lack Ent production (Δ aroB , Δ entC and Δ aroB/ Δ fepA ). On the basis of 8-h broth growth curves in triplicate, we did not observe any significant difference in growth of theses mutants in LB medium ( Supplementary Fig. 5 ). E. coli and its isogenic mutants were plated on chrome azurol S (CAS) plates to detect the expression of the siderophore. This assay is founded on the observation that CAS gives a distinct blue colour when in complex with iron. While iron is chelated by siderophores effectively, an orange halo forms around the siderophore-producing bacteria. As expected, Δ fepA showed a prominent orange-coloured halo, which was much greater than wild-type (WT) E. coli. Also as predicted, no halo formation was observed for Δ aroB, Δ entC ( Fig. 2a ), or Δ aroB/ Δ fepA mutants ( Fig. 3a , upper panel). Overnight-grown Δ fepA (10 6 colony-forming units (CFUs) per ml) produced ∼ 2.5 μg of Ent ( Fig. 2b ), as quantified on CAS agar plates. Importantly, ferric-iron-saturated Ent did not form halos in this assay, confirming that the Ent used in this study was the aferric form ( Fig. 2c ). In addition, the overnight culture supernatants (normalized to equivalent number of bacteria) with or without dipyridyl were tested for MPO inhibitory activity. The iron-depleted bacterial culture supernatant obtained from Δ fepA showed substantial inhibition of MPO activity when compared with WT E. coli , whereas the supernatants obtained from Δ aroB and Δ entC did not exhibit MPO inhibitory activity ( Fig. 2d ). Interestingly, the inhibitory activity of iron-sufficient LB culture supernatants from WT and fepA mutants was modest ( Fig. 2d ). This result suggests that Ent or its precursors secreted into the media may be saturated with the Fe +3 present in the LB media, or that the relatively high iron in LB might repress Fur-mediated biosynthesis of siderophores, specifically of Ent. These findings support the above observation ( Fig. 1c ) that only the apo forms of Ent and DHBA exhibit inhibition of MPO. Similar to Δ fepA , supernatants from an adherent-invasive E. coli strain (LF82) isolated from a Crohn’s disease patient [26] exhibited increased MPO inhibitory activity ( Fig. 2e ). To test the stability of Δ fepA supernatant, we subjected the supernatant to various conditions (24 h at −80 °C, 4 °C, room temperature ( ∼ 25 °C), 37 °C, freeze/thawed three times or boiled for 5 min). With the exception of boiling, Δ fepA supernatant retained its MPO and LPO inhibitory activity after the treatments ( Supplementary Fig. 6 ). 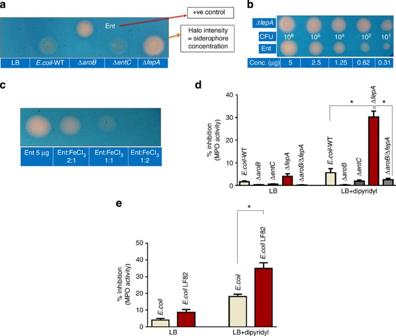Figure 2: Ent-overproducingE. coliexerts more potent MPO inhibitor activity. WTE. coliand its isogenic Ent mutants ΔaroB, ΔentC, ΔfepAand ΔaroB/ΔfepAwere grown overnight in LB and subsequently grown in LB media containing iron chelator 2,2′-dipyridyl (350 μM) for another 6 h. Afterwards, bacteria were pelleted down and supernatants were tested for their MPO inhibitory activity. (a) Representative photograph showing siderophore production on CAS plates by WTE. coliand Ent mutants. (b) Ent-overproducing ΔfepAmutant was plated on CAS plate. Different concentrations of apo-Ent (Sigma) were applied on the CAS plate to quantitate the amount of Ent produced by ΔfepAmutant. (c) Ent saturated with FeCl3in different proportions was plated on the CAS plate. (d) Bar graph displaying the % inhibition of MPO activity by spent media obtained from WTE. colior Ent mutants grown in LB or LB+2,2′-dipyridyl. (e) WT and the adherent-invasiveE. colistrain LF82 were grown as indand the clear supernatants were used to test their MPO inhibitory activity. Results are expressed as mean±s.e.m. and are representative of six independent experiments.*P<0.05, unpairedt-test. Figure 2: Ent-overproducing E. coli exerts more potent MPO inhibitor activity. WT E. coli and its isogenic Ent mutants Δ aroB , Δ entC , Δ fepA and Δ aroB/ Δ fepA were grown overnight in LB and subsequently grown in LB media containing iron chelator 2,2′-dipyridyl (350 μM) for another 6 h. Afterwards, bacteria were pelleted down and supernatants were tested for their MPO inhibitory activity. ( a ) Representative photograph showing siderophore production on CAS plates by WT E. coli and Ent mutants. ( b ) Ent-overproducing Δ fepA mutant was plated on CAS plate. Different concentrations of apo-Ent (Sigma) were applied on the CAS plate to quantitate the amount of Ent produced by Δ fepA mutant. ( c ) Ent saturated with FeCl 3 in different proportions was plated on the CAS plate. ( d ) Bar graph displaying the % inhibition of MPO activity by spent media obtained from WT E. coli or Ent mutants grown in LB or LB+2,2′-dipyridyl. ( e ) WT and the adherent-invasive E. coli strain LF82 were grown as in d and the clear supernatants were used to test their MPO inhibitory activity. Results are expressed as mean±s.e.m. and are representative of six independent experiments. * P <0.05, unpaired t -test. 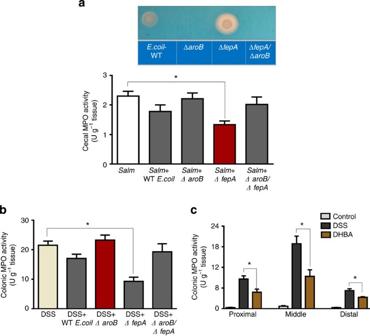Figure 3: Inhibition of MPO activity by Ent and DHBA in experimental colitis. Salmonellaand DSS-induced colitic mice were orally gavaged with overnight-grown WTE. colior Ent mutants (109CFU per mouse,n=4–5). Mice were euthanized via CO2asphyxiation and caecal and colonic MPO activity was subsequently quantified. (a) Caecal MPO, upper panel showing lack of Ent production in ΔaroB/ΔfepAmutant. (b) Colonic (middle portion) tissue samples from the DSS-treated group. (c) DSS-induced colitic mice (n=4) were orally gavaged with DHBA (100 mg kg−1body weight) and after 3 h, mice were euthanized via CO2asphyxiation and MPO activity was quantified in proximal, middle and distal regions of colon. Results are expressed as mean±s.e.m. and are representative of two independent experiments with 4–5 mice per group.*P<0.05, unpairedt-test. Full size image Figure 3: Inhibition of MPO activity by Ent and DHBA in experimental colitis. Salmonella and DSS-induced colitic mice were orally gavaged with overnight-grown WT E. coli or Ent mutants (10 9 CFU per mouse, n =4–5). Mice were euthanized via CO 2 asphyxiation and caecal and colonic MPO activity was subsequently quantified. ( a ) Caecal MPO, upper panel showing lack of Ent production in Δ aroB/ Δ fepA mutant. ( b ) Colonic (middle portion) tissue samples from the DSS-treated group. ( c ) DSS-induced colitic mice ( n =4) were orally gavaged with DHBA (100 mg kg −1 body weight) and after 3 h, mice were euthanized via CO 2 asphyxiation and MPO activity was quantified in proximal, middle and distal regions of colon. Results are expressed as mean±s.e.m. and are representative of two independent experiments with 4–5 mice per group. * P <0.05, unpaired t -test. Full size image Ent-overproducing E. coli inactivates MPO in colitic mice Next, we performed in vivo studies to determine whether introducing Ent mutants to mice with intestinal inflammation would inhibit MPO activity. We employed infectious Salmonella -induced gastroenteritis and chemical colitogen dextran sulfate sodium (DSS)-induced colitis models, which are characterized by caecal and colonic inflammation, respectively. As shown in our previous studies [27] , [28] , Salmonella -induced gastroenteritis in mice pretreated with streptomycin exhibited caecal emptying and shrinkage. Mice with caecal inflammation inoculated with WT E. coli or its isogenic mutants Δ fepA or Δ aroB did not show significant alterations in inflammatory cell infiltrate or caecal pathology, as determined with haematoxylin and eosin staining of caecal sections ( Supplementary Fig. 7A ). Similarly, colonic pathology and infiltration of macrophages were unaltered in mice that received WT E. coli or its isogenic mutants Δ fepA or Δ aroB/ Δ fepA when compared with control animals (given DSS alone) in the experimental model of DSS-induced acute colitis ( Supplementary Fig. 7B,C ). Salmonella -given mice that were inoculated with WT E. coli or Δ fepA , but not Δ aroB or Δ aroB/ Δ fepA , demonstrated a consistent reduction in caecal MPO activity when compared with control mice given Salmonella alone ( Fig. 3a ). Likewise, mice given WT E. coli or Δ fepA , but not Δ aroB or Δ aroB/ Δ fepA , presented with a significant reduction in colonic MPO levels in the DSS-induced colitis model ( Fig. 3b ). Further, orally administered DHBA also substantially reduced MPO activity in all three regions of the colon (proximal, middle and distal) of DSS-treated mice ( Fig. 3c ). These results indicate that Ent can inhibit MPO activity in colitic mice whether generated in vivo by E. coli or administered orally. Ent provides survival advantage to E. coli in the inflamed gut To evaluate whether Ent-induced inhibition of MPO confers a survival advantage to E. coli in vitro by limiting generation of the bactericide hypohalous acid [10] , we measured the viability of WT E. coli exposed to MPO–H 2 O 2 in the presence or absence of Ent or DHBA. As shown in Fig. 4a,b , Ent and DHBA substantially reduced the bactericidal activity of MPO–H 2 O 2 . Notably, Fe +3 -bound Ent or DHBA (1:1 stoichiometric ratio) failed to prevent MPO–H 2 O 2 -mediated bacterial killing ( Fig. 4b ), confirming our previous observation that the aferric form of Ent is required for inhibition of MPO activity. Both Ent and DHBA rescued bacteria from LPO–H 2 O 2 -mediated killing ( Supplementary Fig. 8 ). To evaluate the effect of MPO–H 2 O 2 on killing bacteria that either lack or overproduce Ent, we exposed WT E. coli and the Ent mutants, Δ aroB , Δ fepA and Δ aroB/ Δ fepA , to MPO–H 2 O 2 . The Ent-overproducing E. coli mutant Δ fepA was substantially protected from MPO–H 2 O 2 -induced bacterial killing ( Fig. 4c ) compared with WT E. coli and the Ent-deficient Δ aroB and Δ aroB/ Δ fepA mutants, which survived poorly ( Fig. 4c ). Moreover, supernatants from the Δ fepA mutant grown in iron-depleted LB substantially rescued Δ aroB from MPO–H 2 O 2 -induced killing ( Fig. 4d ), whereas supernatants from Δ aroB/ Δ fepA mutants offered no protection, suggesting that Ent released in the media from Δ fepA might protect Δ aroB against MPO-mediated bacterial killing. 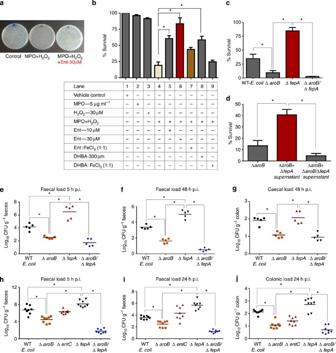Figure 4: Ent provides survival advantage toE. coli in vitroand in the inflamed gutin vivo. Overnight-grown WTE. coliin LB medium was resuspended in PBS and then incubated with MPO (5 μg ml−1) and H2O2(30 μM) with or without Ent (30 μM) or DHBA (300 μM) for 30 min. (a) Image displays overnight-grown bacterial colonies on an agar plate. (b) Bar graph representing % survival of WTE. coliunder different treatment. WTE. coli, ΔaroBand ΔfepAmutants were grown in an iron-depleted medium for 6 h and subsequently examined for MPO–H2O2-mediated bacterial killing as described above. (c) Bar graph represents % survival of WTE. coli, ΔaroB, ΔfepA andΔaroB/ΔfepAmutants. (d) Effect of ΔfepAand ΔaroB/ΔfepAculture supernatant on survival of ΔaroB. (e–j) Streptomycin-pretreatedSalmonella-induced gastroenteritis mice (n=5) orally gavaged with WTE. coli, ΔaroB, ΔfepAor ΔaroB/ΔfepAmutants (1.0 × 108CFU per mouse). Faecal CFUs were quantified on selective (kanamycin 30 μg ml−1) agar plates. Dot plot represents faecal shedding ofE. colimutants from theSalmonella-induced gastroenteritis model after (e) 5 and (f) 48 h. (g) Caecal bacterial load at 48 h. Mice (n=8) exhibiting symptoms of DSS-induced colonic inflammation were orally gavaged with 10 × 109CFU of ΔaroB, ΔentC, ΔfepAor ΔaroB/ΔfepAmutants. Faecal shedding and colonic tissue loads ofE. colimutants were selectively quantified on kanamycin (30 μg ml−1) agar plates. Dot plot represents faecal shedding ofE. colimutants from DSS-induced colitic mice after (h) 5 h and (i) 24 h. (j) Colonic tissue load after 24 h. Results are expressed as mean±s.e.m. and are representative of two independent mice experiments.In vitroexperiments are representative of four independent experiments. *P<0.05, unpairedt-test. Figure 4: Ent provides survival advantage to E. coli in vitro and in the inflamed gut in vivo . Overnight-grown WT E. coli in LB medium was resuspended in PBS and then incubated with MPO (5 μg ml −1 ) and H 2 O 2 (30 μM) with or without Ent (30 μM) or DHBA (300 μM) for 30 min. ( a ) Image displays overnight-grown bacterial colonies on an agar plate. ( b ) Bar graph representing % survival of WT E. coli under different treatment. WT E. coli , Δ aroB and Δ fepA mutants were grown in an iron-depleted medium for 6 h and subsequently examined for MPO–H 2 O 2 -mediated bacterial killing as described above. ( c ) Bar graph represents % survival of WT E. coli , Δ aroB , Δ fepA and Δ aroB/ Δ fepA mutants. ( d ) Effect of Δ fepA and Δ aroB/ Δ fepA culture supernatant on survival of Δ aroB . ( e – j ) Streptomycin-pretreated Salmonella- induced gastroenteritis mice ( n =5) orally gavaged with WT E. coli , Δ aroB , Δ fepA or Δ aroB/ Δ fepA mutants (1.0 × 10 8 CFU per mouse). Faecal CFUs were quantified on selective (kanamycin 30 μg ml −1 ) agar plates. Dot plot represents faecal shedding of E. coli mutants from the Salmonella- induced gastroenteritis model after ( e ) 5 and ( f ) 48 h. ( g ) Caecal bacterial load at 48 h. Mice ( n =8) exhibiting symptoms of DSS-induced colonic inflammation were orally gavaged with 10 × 10 9 CFU of Δ aroB , Δ entC , Δ fepA or Δ aroB/ Δ fepA mutants. Faecal shedding and colonic tissue loads of E. coli mutants were selectively quantified on kanamycin (30 μg ml −1 ) agar plates. Dot plot represents faecal shedding of E. coli mutants from DSS-induced colitic mice after ( h ) 5 h and ( i ) 24 h. ( j ) Colonic tissue load after 24 h. Results are expressed as mean±s.e.m. and are representative of two independent mice experiments. In vitro experiments are representative of four independent experiments. * P <0.05, unpaired t -test. Full size image We further investigated the extent to which Ent-mediated inhibition of MPO activity protects bacteria in vivo and offers a survival advantage in the inflamed gut. On the basis of the in vitro studies, we hypothesized that the Ent-overproducing Δ fepA mutant, but not the Δ aroB , Δ entC or Δ aroB/ Δ fepA mutants, would demonstrate an in vivo survival advantage in the inflamed gut. After oral gavage of bacteria to mice with robust caecal inflammation in Salmonella gastroenteritis and the DSS-induced colonic inflammation model, we monitored faecal shedding and tissue loads of mutant bacteria. We observed a significant increase in faecal shedding of Δ fepA mutants relative to WT E. coli , Δ entC , Δ aroB and Δ aroB/ Δ fepA mutants ( Fig. 4e,f,h,i ), suggesting that Ent-null mutants were either killed while passing through the intestine or better colonized the inflamed intestinal tract. To distinguish between these two possibilities, we quantified caecal and colonic loads of these Ent mutants. The Ent-overproducing Δ fepA mutant superiorly colonized in the caecal ( Fig. 4g ) and colonic tissue ( Fig. 4j ) compared with the Ent mutants. Taken together, these results indicate that E. coli overproducing Ent survive and colonize better in inflamed colons than do mutants lacking Ent. Lcn2 abrogates Ent-mediated inhibition of MPO activity Having established that MPO secreted by neutrophil granules at the site of infection is vulnerable to inactivation by bacterial siderophores, we next sought to identify potential host proteins that may counter Ent-mediated MPO inactivation. Lcn2, a host siderophore-binding protein present in specific granules of neutrophils, is additionally produced by gut epithelial cells during inflammation [27] , [29] , [30] . To test the possibility that Lcn2 can counter Ent-mediated MPO inhibition, we performed an MPO assay in which Ent or DHBA was pre-incubated with recombinant human or mouse-Lcn2 (siderophore- and iron free). Notably, both human and mouse Lcn2-treated Ent and DHBA failed to inhibit MPO ( Fig. 5a ) and LPO activity ( Fig. 5b ). Together, these results suggest that MPO may be at risk for inactivation by bacterial siderophores upon discharge by neutrophils at the site of infection. However, Lcn2 can rescue MPO from bacterial siderophores, therefore restoring its bactericidal capabilities. 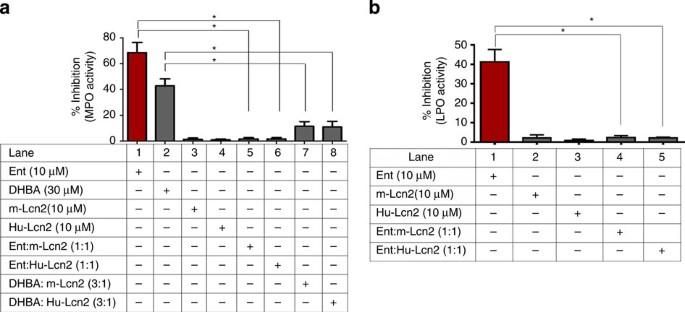Figure 5: Ent bound to Hu-Lcn2 or mouse-Lcn2 failed to inhibit MPO activity. Ent (10 μM) or DHBA (30 μM) was pre-incubated with or without Hu-Lcn2 (10 μM) or mouse-Lcn2 (10 μM) for 3 min and the resulting complex was subsequently incubated with MPO (100 mU) or LPO (50 μg ml−1) for 10 min. After binding to Hu-Lcn2 or mouse-Lcn2, Ent and DHBA failed to inhibit MPO (a) or LPO (b) activity. Results are expressed as mean±s.e.m. and are representative of three independent experiments. *P<0.05, unpairedt-test. Figure 5: Ent bound to Hu-Lcn2 or mouse-Lcn2 failed to inhibit MPO activity. Ent (10 μM) or DHBA (30 μM) was pre-incubated with or without Hu-Lcn2 (10 μM) or mouse-Lcn2 (10 μM) for 3 min and the resulting complex was subsequently incubated with MPO (100 mU) or LPO (50 μg ml −1 ) for 10 min. After binding to Hu-Lcn2 or mouse-Lcn2, Ent and DHBA failed to inhibit MPO ( a ) or LPO ( b ) activity. Results are expressed as mean±s.e.m. and are representative of three independent experiments. * P <0.05, unpaired t -test. Full size image Microbiotal dysbiosis is commonly associated with IBD and is characterized by a bloom in bacterial species belonging to phylum proteobacteria such as E. coli , a typically innocuous resident of the gastrointestinal tract. For instance, Enterobacteriaceae represent 86% of the total bacterial community in ileal Crohn’s disease patients [31] . In this study, we demonstrate a novel survival mechanism in which siderophores expressed by E. coli can inhibit the host’s potent neutrophilic antibacterial enzyme MPO in a dose-dependent fashion. Such inhibition of MPO requires iron-free Ent and DHBA. By spectral analysis, we provide evidence that Ent and DHBA divert the peroxidase from the halogenation cycle by acting as potent suicide substrates of the peroxidase-catalysed reaction. The E. coli mutant (Δ fepA ), which overproduces Ent, exhibits greater MPO inhibitory activity and colonizes the inflamed mouse intestine better than mutants that completely lack Ent expression ( aroB ). The host’s siderophore-binding protein, Lcn2, can inhibit Ent- and DHBA-mediated MPO inhibition, thereby neutralizing the E. coli survival advantage. IBDs are characterized by an elevated innate immune response accompanied by generation of reactive oxygen species (ROS) and nitric oxide radicals. To survive in the chemically hostile environment, E. coli or the microbiota must be equipped with endogenous machinery or molecules that can effectively neutralize host-derived pro-oxidants. Accordingly, several studies have demonstrated that bacterial siderophores can act as ROS-neutralizing agents [32] , [33] , [34] . Recently, Adler et al. demonstrated that an entE mutant strain impaired in Ent production was unable to form colonies on M9 agar medium; however, addition of Ent or ascorbate rescued the mutant. Their study also demonstrated that Ent-Fe +3 hydrolysis in the cell cytoplasm not only fulfills iron needs, but also provides the cell with a molecule rich in hydroxyl groups that can scavenge ROS [35] . The same group previously demonstrated that Ent is necessary to protect E. coli against pyochelin, a siderophore from P. aeruginosa -induced oxidative stress [36] . Thus, in addition to helping E. coli acquire iron, Ent may also grant protection in an oxidizing environment in several ways. Being rich in –OH groups, Ent could neutralize external host-derived oxidative damage-inducing molecules. Further, Ent may also serve as an endogenous antioxidant to the bacterium when iron is internalized. Finally, Ent could reduce iron availability to immune cells, which require iron to produce hydroxyl radicals via the Haber–Weiss reaction. Our study supports the notion of Ent protecting against oxidative stress, but in a new dimension: through blocking the production of the potent oxidizing agent hypohalous acid. Notably, both salmochelin (glycosylated enterobactin) and non-catecholate siderophores (that is, yersiniabactin and ferrichrome) failed to inhibit MPO activity at concentrations even higher than Ent. This result suggests that MPO activity is specifically inhibited by Ent. Neutrophils are the richest source of Lcn2 (ref. 37 ). It has been shown that mucosal Lcn2 exhibits pro-inflammatory and iron-sequestering activity in response to Ent [38] . Specifically, Ent-bound Lcn2 can activate mucosal epithelia to secrete interleukin-8, a potent neutrophil chemotactic agent. Thus, Lcn2 represents a novel mechanism of sensing microbial metabolites to modulate the host immune response. Accordingly, mice lacking Lcn2 are sensitive to E. coli infections [39] , [40] . Consistent with these results, our study indicates that the pro-inflammatory activity of Lcn2 could be also due to its ability to bind Ent and preserve MPO activity, ultimately resulting in a heightened inflammatory response mediated by hypohalous acid via generation of ROS [41] . Acquiring iron from the host represents a major challenge for bacterial aerobic metabolism and growth. Bacteria overcome this limitation by producing siderophores, which have high affinity for iron. Further, inflammatory diseases, IBD in particular, are associated with a low iron environment or anaemia due to upregulation of hepcidin and/or increased expression of iron-sequestering proteins [42] , [43] . As such, the iron-depleted environment may signal or impose selective pressures on E. coli to produce higher levels of Ent or modified siderophores. These siderophores not only help in acquiring iron but may also function as MPO inhibitors. Our study suggests that the host’s innate immune protein Lcn2, which can bind Ent and prevent MPO inhibition, may exert immune pressure on E. coli to express altered and stealth siderophores. For example, E. coli is known to express altered stealth siderophores such as salmochelin and yersiniabactin, which display increased iron-scavenging activity, thereby favouring bacterial growth and limiting the availability of iron to immune cells [44] . These stealth siderophores are known to avoid recognition by Lcn2, which may grant the bacteria superior survival in the inflamed environment. Crouch et al. [45] showed that Salmonella synthesizes approximately equal amounts of enterobactin and salmochelin. On a molar ratio, Salmonella may have less enterobactin compared with E. coli and consequently exhibited reduced MPO inhibitory activity, because both enterobactin and salmochelin are products of the same pathway. Herein, we demonstrate that salmochelin fails to inhibit MPO activity. In addition, Salmonella and certain clinical isolates of E. coli are known to convert the cyclic enterobactin to linearized enterobactin [46] , [47] . However, it is unclear whether linearized enterobactin avoids Lcn2 recognition or displays altered MPO inhibitory activity. The flexibility of E. coli in expressing multiple and independent siderophores may explain its success as an opportunistic pathogen in extraintestinal tissues and in the evolution of several E. coli pathotypes of major public health concern [48] . Taken together, our study demonstrates that the E. coli siderophore Ent and its monomeric form DHBA inhibit MPO activity by acting as suicidal substrates, providing a distinct survival advantage to E. coli in the inflamed gut. Thus, E. coli siderophores serve as dual-purpose molecules, both in iron acquisition and in protection from oxidative stress imposed by host innate immunity. Further, the neutralization of Ent-mediated inhibition of MPO activity by Lcn2 may exert selective immune pressure on E. coli to evolve and synthesize stealth siderophores (for example, aerobactin and yersiniabactin), which resist chelation by host Lcn2. Moreover, the interplay between siderophores and host innate immunity may result in the altered metagenomics, which could be a potential mechanism for the E. coli bloom in IBD. Our study also suggests that Ent may interfere with other Fe +3 -dependent ROS-generating enzymes (for example, NADPH oxidases) [49] and overall reduce the oxidative stress imposed by the host innate immunity. Future studies with MPO-deficient mice are warranted to convincingly demonstrate to what extent enterobactin–MPO interaction dictates E. coli survival. It is interesting to note that E. coli Nissle 1917, a member of the family Enterobacteriaceae , encodes four siderophores including Ent, salmochelin, aerobactin and yersiniabactin [44] . This strain, also known as ‘Mutaflor’, has been used in Germany for many years to treat colitis [50] and constipation [51] . In the same line, this study may facilitate further investigation of the utility of siderophore-based molecules to target MPO, a culprit in the generation of deleterious oxidatively modified biomolecules, which play a critical role in multiple chronic diseases [52] . In conclusion, as schematically represented in Fig. 6 , we have demonstrated that siderophores generated by E. coli , by virtue of inhibiting the MPO-catalysed reaction with H 2 O 2 , define a new defence mechanism of microbiotal warfare against the host innate immune system. 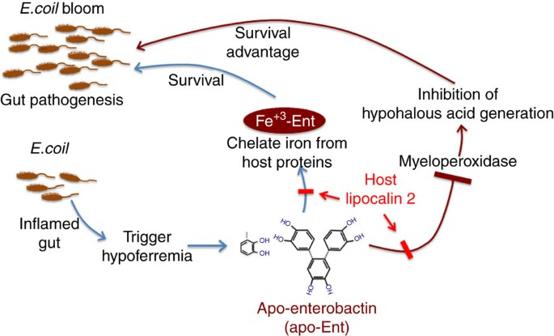Figure 6: Potential mechanism by which Ent-mediated MPO inhibition provides a survival advantage toE. coliin the inflamed intestine. Hypoferremia in the inflamed gut signals bacteria (E. coli) to produce more enterobactin (Ent), which not only helps to efficiently acquire iron from the environment but also inactivates host antibacterial enzyme myeloperoxidase (MPO). The dual activities of Ent provide a survival advantage despite the inflammatory milieu, resulting inE. colibloom. The inhibition of MPO activity by Ent is counter-regulated by host siderophore-binding protein, Lipocalin 2. Figure 6: Potential mechanism by which Ent-mediated MPO inhibition provides a survival advantage to E. coli in the inflamed intestine. Hypoferremia in the inflamed gut signals bacteria ( E. coli ) to produce more enterobactin (Ent), which not only helps to efficiently acquire iron from the environment but also inactivates host antibacterial enzyme myeloperoxidase (MPO). The dual activities of Ent provide a survival advantage despite the inflammatory milieu, resulting in E. coli bloom. The inhibition of MPO activity by Ent is counter-regulated by host siderophore-binding protein, Lipocalin 2. Full size image Reagents Human MPO, iron-free Ent, ferric chloride, hydrogen peroxide, O -dianisidine hydrochloride, DHBA, ABAH, dimethyl sulfoxide, ferrichrome and 2,2′ dipyridyl were procured from Sigma (St Louis, MO). Yersiniabactin (ybt) and salmochelin S4 were obtained from EMC microcollections (GmbH, Germany). Bovine milk LPO was purchased from Worthington Biochemical Corp., (Lakewood, NJ). Guaiacol (2-methoxyphenol) was obtained from Alfa Aesar (MA, USA). Human Lcn2 (also known as neutrophil gelatinase-associated lipocalin), murine Lcn2 (also known as 24p3) and human MPO were purchased from R&D Systems (Minneapolis, MN). The commercially available recombinant Lcn2 proteins were free of endotoxin, siderophore and iron. E. coli and its isogenic siderophore mutants WT E. coli (EcK12) and its isogenic mutant of 3-dehydroquinate synthase ( Δ aroB) were obtained from The E. coli Genetic Stock Center, Yale University. WT and its isogenic isochorismate synthase 1 ( Δ entC) , ferrienterobactin permease ( Δ fepA) and aroB-fepA double mutants (Δ aroB/ Δ fepA) were gifts from Dr Kathleen Postle, Pennsylvania State University. The EcK12 strain has been shown to colonize poorly in the murine intestinal tract [53] and is incapable of disseminating to extraintestinal tissues, such as the spleen, liver and mesenteric lymph nodes [54] . Bacterial cultures Non-pathogenic WT E. coli and its isogenic Ent mutants (Δ entC , Δ aroB , Δ fepA and Δ aroB/ Δ fepA ) were grown in LB media overnight at 37 °C. 2,2′-dipyridyl (350 μM), which complexes with transition metals, was added to make the LB media iron deficient. The bacteria were pelleted and grown in LB media with or without 2,2′-dipyridyl for 6 h [38] . The bacterial CFUs were adjusted based on the optical density at 600 nm. Media containing an equal number of bacteria were centrifuged and clear supernatants were used for the in vitro MPO and LPO activity assay. Mice Balb/c mice were bred and maintained at the animal house facility at the Pennsylvania State University. Animal experimental protocols were approved by the Pennsylvania State University IACUC committee. MPO and LPO assay Human MPO (50 U mg −1 protein) was reconstituted with 0.1 M potassium phosphate buffer (pH 6.0) and stored at −80 °C. Aferric Ent was reconstituted in dimethyl sulfoxide and stored at −80 °C. DHBA was reconstituted in PBS (pH 8.0). Salmochelin was reconstituted in water and yersiniabactin was dissolved in methanol. Assays were carried out in 96-well plates (Corning) in triplicate with appropriate vehicles/buffers throughout the study. This method is based on the principle that MPO oxidizes guaiacol in the presence of H 2 O 2 to chromophore 3,3′-dimethoxy-4, 4′-biphenylquinone [55] . Briefly, MPO (100 mU, final concentration) or LPO (50 μg ml −1 , final concentration) were pre-incubated with vehicle/appropriate buffers, various concentrations of siderophores or indicated molecules for 10 min. The reaction was initiated by adding final concentrations of 100 mM guaiacol and 6.7 × 10 −3 % H 2 O 2 . The change in absorbance at 470 nm was measured over a period of 20 min at 1-min intervals. One unit of MPO activity was defined as the amount that degraded 1.0 μmol of peroxidase per minute at 25 °C. As a positive control, an MPO inhibitor, ABAH was used at half-maximal inhibitory concentration of 16 μM in all of the experiments. We also used MPO oxidized by O -dianisidine-HCl in the presence of H 2 O 2 (ref. 56 ) and observed similar results. The data presented in this study employed the guaiacol method, as it was found to be more sensitive than O -dianisidine. CAS assay for Ent-secreting E. coli mutants CAS agar plates were prepared according to the protocol as outlined in ref. 57 . Briefly, overnight bacterial cultures grown in LB media were placed on CAS agar plates, incubated overnight at 37 °C and monitored for orange-coloured halo formation. CAS gives a distinctive blue colour when in complex with iron. When the iron is instead chelated by bacterial siderophores, orange halos develop around the siderophore-producing bacteria. The intensity of halo formation is directly proportional to the concentration of siderophores secreted by the bacteria. Purified Ent (Sigma) was used as a positive control. In vitro bacterial killing assay The in vitro bacterial killing assay was performed as described by Atosuo and Lilius [58] . Briefly, the MPO reaction mixture was prepared by first adding the MPO (5.0 μg ml −1 , R&D systems) with or without Ent (10 or 30 μM) or DHBA (300 μM) at final concentrations in sterile conditions. Hydrogen peroxide (30 μM) was then added to the reaction mixture and incubated at room temperature for 5 min. Finally, WT or Ent mutant bacteria grown overnight at 37 °C with 250 r.p.m. shaking (2 × 10 6 CFU ml −1 ) were added to the reaction mixture. In some experiments, Ent (10 μM) or DHBA (30 μM) was incubated with 10 μM of Hu-Lcn2 or murine Lcn2 before being added to the reaction mixture. After 30 min of incubation at room temperature, the reaction mixture was serially diluted and plated on non-selective LB plates in triplicates. Plates were incubated overnight at 37 °C and bacterial CFU on plates were quantified. Streptomycin-pretreated Salmonella -induced gastroenteritis Eight-week-old Balb/c female mice were pretreated with streptomycin orally and subsequently infected with Salmonella to induce colitis as described previously [27] . On the day of the experiment, water and food were withdrawn 4 h before treatment and 20 mg of streptomycin in 100 μl of sterile water was administered by oral gavage. Afterwards, animals were supplied with water and food ad libitum . At 20 h after streptomycin treatment, water and food were withdrawn again for 4 h before the mice were orally administered 10 8 CFU per mouse of Salmonella enterica serovar Typhimurium (SL3201) followed by 10 8 CFU per mouse E. coli Ent mutants, and were subsequently euthanized at 48 h. Thoroughly washed caeca (free from faecal matter) were used for the MPO activity assay as described above. DSS-induced colitis in mice Eight-week-old female Balb/c mice ( n =4–5) were administered 2.5% DSS (MP Biomedicals) in drinking water over a period of 7 days [59] . Induction of colonic inflammation was confirmed via faecal occult blood, diarrhoea and loss in body weight. Mice were orally inoculated (1 × 10 9 CFU per mouse) with WT E. coli or its isogenic Ent mutants Δ aroB , Δ entC (lacks Ent expression), Δ fep A (overproduces Ent) or Δ aroB/ Δ fep A (lacks Ent expression). In another set of experiments, DSS-induced colitic mice were orally administered DHBA (100 mg kg −1 body weight in 0.1 ml of 5% NaHCO 3 ) [60] . Five hours after administration of either bacteria or 3 h after DHBA, mice were euthanized via CO 2 asphyxiation, and colons were harvested for the MPO activity assay. Briefly, colons were homogenized in 0.5% cetyltrimethyl ammonium bromide (Sigma) in potassium buffer (pH 6.0), freeze–thawed three times, sonicated and centrifuged. The MPO assay was performed in the clear supernatants as described above. In vivo survival and colonization assay Eight-week-old female Balb/c mice ( n =4–5) were administered 2.5% DSS (MP Biomedicals) in drinking water [59] . Induction of colonic inflammation was confirmed via faecal occult blood and loss in body weight. On day 5 of DSS treatment, mice were administered streptomycin (20 mg per mouse) and after 24 h, orally gavaged (10 × 10 9 CFU per mouse) with either Δ aroB or Δ entC (lacks Ent expression) or Δ fep A (overproduces Ent) mutants. DSS was restricted to 5 days because mice treated with DSS for 7 days exhibited severe diarrhoea. Faecal shedding of bacteria was measured 5 and 24 h post inoculation using selective agar plates (kanamycin 30 μg ml −1 ). After 24 h, mice were euthanized via CO 2 asphyxiation. Colons were flushed gently with PBS to remove faecal matter, homogenized and used to quantitate the colonization of mutant bacteria on selective agar plates as described above. Spectral analysis Basal spectra were recorded at 412 nm for freshly reconstituted LPO (2.6 nM) in phosphate buffer (0.1 M). Spectral analysis of LPO during the oxidation of Ent, DHBA and ABAH was recorded at 412 nm using CARY50BIO UV-Visible Spectrophotometer. Briefly, LPO was incubated with either Ent, DHBA or ABAH (1, 10 or 30 μM, respectively) for 1 min. The reaction was started by the addition of 30 μM H 2 O 2 . The spectra were recorded every 10 s. Each spectrum is an average of three scans taken in 1.0 s [24] . Histology and immunohistochemistry analysis At termination of the experiment, caecum and colonic tissue were isolated and preserved in 10% buffered formalin solution for 24 h. Caeca of all groups were processed for paraffin embedding and serial paraffin sections (5 μm) were collected and stained with haematoxylin and eosin. Colons obtained from different groups were frozen as Swiss roll in optimum cutting temperature (OCT, Tissue-Tek) compound for cryostat sectioning. Immunoreactivity to colonic macrophages was revealed using rat anti-mouse F4/80 antibody, clone Cl:A3-1 (1:50 dilution, AbD Serotec) as described earlier [61] . An appropriate negative isotype control (rat IgG2b) was included to omit nonspecific staining. Statistical analysis All experimental results were reproduced in at least three independent experiments performed in triplicate. Results are expressed as means with their s.e. Significance of difference between groups was analysed by an unpaired t -test using GraphPad Prism software 6.0. A P value less than 0.05 was considered statistically significant. How to cite this article: Singh, V. et al. Interplay between enterobactin, myeloperoxidase and lipocalin 2 regulates E. coli survival in the inflamed gut. Nat. Commun. 6:7113 doi: 10.1038/ncomms8113 (2015).